MED26 regulates the transcription of snRNA genes through the recruitment of little elongation complex Regulation of transcription elongation by RNA polymerase II (Pol II) is a key regulatory step in gene transcription. Recently, the little elongation complex (LEC)—which contains the transcription elongation factor ELL/EAF—was found to be required for the transcription of Pol II-dependent small nuclear RNA ( snRNA ) genes. Here we show that the human Mediator subunit MED26 plays a role in the recruitment of LEC to a subset of snRNA genes through direct interaction of EAF and the N-terminal domain (NTD) of MED26. Loss of MED26 in cells decreases the occupancy of LEC at a subset of snRNA genes and results in a reduction in their transcription. Our results suggest that the MED26-NTD functions as a molecular switch in the exchange of TBP-associated factor 7 (TAF7) for LEC to facilitate the transition from initiation to elongation during transcription of a subset of snRNA genes. Transcription by RNA polymerase II (Pol II) proceeds through multiple stages, beginning with recruitment of Pol II and other components of the transcription apparatus to the promoter to form a pre-initiation complex, followed by ATP-dependent unwinding of the DNA template and transcription initiation. Following initiation, Pol II moves away from the promoter, leading to establishment of a productive elongation complex that can complete synthesis of the nascent transcript. Although research for many years was mainly focused on mechanisms that control the pre-initiation and initiation stages of transcription [1] , [2] , [3] , a growing body of evidence indicates that transcription of many genes is also regulated during transcription elongation [4] , [5] . The product of the members of the eleven-nineteen lysine-rich leukaemia ( ELL ) gene, which is a translocation partner of mixed lineage leukaemia, and its binding partner ELL-associated factors (EAFs) are key regulators of transcription elongation by Pol II [6] , [7] . Recently, two distinct ELL/EAF-containing complexes, super elongation complex (SEC) and little elongation complex (LEC), have been identified. SEC contains P-TEFb (positive transcription elongation factor), ELL/EAF and additional factors, mixed lineage leukaemia-fusion partner proteins [8] , [9] , [10] , and it regulates transcription elongation of a variety of protein-coding genes, including c-Myc , Hsp70 , Hox and HIV provirus [11] . LEC contains ELL/EAF and additional components, KIAA0947 and NMDA receptor regulated 2 (NARG2), which were also identified as components of Drosophila LEC and are called ICE1 and ICE2 (interacts with carboxy terminus of ELL), respectively [12] . Recently, it was shown that LEC specifically regulates the transcription of Pol II-transcribed small nuclear RNA ( snRNA ) genes [12] , [13] . Pol II-transcribed snRNA genes are structurally different from Pol II-transcribed protein-coding genes [14] . The promoter is composed of a proximal sequence element and an enhancer-like distal sequence element. In addition, Pol II-transcribed snRNA genes contain a 3′ box instead of a polyadenylation signal, which is required for 3′ end formation [15] . Transcription of Pol II-transcribed snRNA genes requires an integrator complex that specifically binds to the Ser7-phosphorylated form of the Pol II C-terminal domain (CTD) and proceeds to the 3′ end formation [16] , [17] . Inhibitors of P-TEFb reduce the 3′-box-dependent 3′ end processing but do not affect transcription elongation of the snRNA genes [18] , indicating that there is different regulation of transcription elongation between Pol II-dependent protein-coding genes and snRNA genes. Mediator is an evolutionarily conserved transcriptional coregulatory complex that is needed for the relay of regulatory signals between gene-specific transcription activators and the basal initiation machinery [19] . Recently, it has been shown that Mediator is involved in the activation of transcription of a number of Pol II-dependent genes at multiple steps, including pre-initiation, promoter clearance, transcription elongation, transcription termination and mRNA splicing steps [20] , [21] , [22] , [23] , [24] . In metazoans, Mediator is composed of ~30 distinct subunits and exists in multiple and functionally distinct forms that share common core subunits, which are distinguished by the presence or absence of a kinase module composed of cyclin C, CDK8, MED12 and MED13 (ref. 25 ). Notably, a subset of Mediator contains an additional subunit, MED26. MED26-containing Mediator is copurified with only a small amount of a kinase module but with sub-stoichiometric Pol II, and it plays an important role in gene activation [25] , [26] , [27] . The amino-terminal domain (NTD) of MED26 is the most highly conserved region of MED26 and is similar to the NTDs of the elongation factors TFIIS and elongin A [28] , [29] . Previously, we found that MED26-NTD copurifies with two ELL/EAF-containing complexes, SEC and LEC [20] . We showed that MED26-NTD contributes to recruitment of SEC to a subset of human protein-coding genes including c-Myc and Hsp70 through direct interaction of MED26-NTD with EAF [20] . However, generality of the role of MED26 in recruiting ELL/EAF-containing complexes has not been established. Here we present evidence that the human Mediator subunit MED26 plays a role in the recruitment of LEC to a subset of Pol II-transcribed snRNA genes through direct interaction of EAF and MED26-NTD. Depletion of MED26 in cells decreases the occupancy of LEC at a subset of snRNA genes and results in reduction of expression of the genes. In addition, we identified the MED26-NTD-binding region of EAF1. Intriguingly, we found that there is a partially similar amino-acid sequence in EAF and TATA-binding protein (TBP)-associated factor 7 (TAF7) and that each of the regions is necessary for direct interaction with MED26-NTD. TAF7 has been shown to repress the initiation or post-initiation process of transcription by preventing premature transcription initiation or elongation in a transcription factor IID (TFIID)-dependent or -independent manner [30] , [31] . Our results indicate that TAF7 directly interacts with MED26-NTD and blocks LEC recruitment to a subset of snRNA genes. On the basis of our findings, we propose a model in which MED26-NTD functions as a molecular switch that interacts with TAF7 in the initiation process and then exchanges it for LEC to facilitate the transition from initiation to elongation during transcription of a subset of snRNA genes. NTD of MED26 is required for interaction with LEC Since previous mass spectrometric analysis indicated that MED26-NTD interacts with LEC [20] , we performed western blot to determine whether MED26-NTD is critical for LEC interaction with Mediator. We purified Mediator from HeLa S3 cells stably expressing FLAG-MED26 wild type (wt) or a MED26-NTD deletion mutant (C-terminal short (CS): 421–600). Mediator purified through FLAG-MED26-wt or MED26-CS was copurified with Pol II and Mediator components; however, deletion of MED26-NTD resulted in loss of Mediator interaction with LEC components, ICE1 (KIAA0947), ELL and EAF1 ( Fig. 1a ). Since we previously showed that substitution of two amino-acid residues R61 and K62 of MED26-NTD with A interferes with both direct interaction with EAF and interaction with the components of SEC in cells [20] , we tested whether the same substitution interferes with the interaction of MED26-NTD and LEC in cells. FLAG-MED26-wt was copurified with LEC, but MED26-R61A, K62A was not ( Fig. 1b ). These results show that MED26-NTD is critical for interaction of Mediator with LEC. In turn, we tested whether LEC is copurified with MED26-containing Mediator. We purified LEC from 293FRT cells stably expressing FLAG-ICE2 (NARG2). FLAG-ICE2 was copurified with Mediator subunits MED26 and MED1, in addition to ICE1, ELL and EAF1 ( Fig. 1c ), but FLAG-BTBD19 was not copurified with any of these proteins ( Fig. 1c ), indicating that LEC interacts with MED26-containing Mediator. Taken together, the results indicate that MED26-NTD functions as a docking site for LEC to recruit it to Mediator. 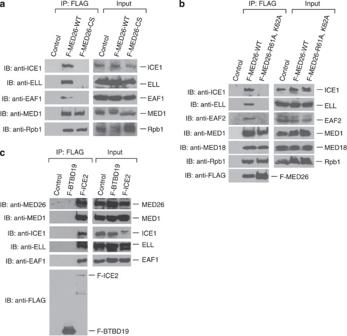Figure 1: Association of MED26-NTD with LEC. (a) Western blot for FLAG-immunopurified complexes from parental HeLa cells (control) and HeLa cells stably expressing FLAG-tagged MED26 wt and N-terminal deletion mutant (CS: 421–600). (b) Western blot for FLAG-immunopurified complexes from parental HeLa cells (control) and HeLa cells stably expressing FLAG-tagged MED26 wt and point mutant (R61A, K62A). (c) Western blot for FLAG-immunopurified complexes from parental 293FRT cells (control) and 293FRT cells stably expressing FLAG-tagged BTBD19 and FLAG-tagged ICE2 (NARG2). Figure 1: Association of MED26-NTD with LEC. ( a ) Western blot for FLAG-immunopurified complexes from parental HeLa cells (control) and HeLa cells stably expressing FLAG-tagged MED26 wt and N-terminal deletion mutant (CS: 421–600). ( b ) Western blot for FLAG-immunopurified complexes from parental HeLa cells (control) and HeLa cells stably expressing FLAG-tagged MED26 wt and point mutant (R61A, K62A). ( c ) Western blot for FLAG-immunopurified complexes from parental 293FRT cells (control) and 293FRT cells stably expressing FLAG-tagged BTBD19 and FLAG-tagged ICE2 (NARG2). Full size image Purification and reconstitution of LEC To address the interactions of individual factors within LEC, we expressed FLAG-ICE2, HA-ICE1, HA-ELL and Myc-EAF1 in the indicated combinations using a baculovirus expression system. FLAG-ICE2 was copurified with HA-ELL only in the presence of HA-ICE1 ( Fig. 2a ), indicating that ICE1 is required for formation of the protein complex containing ICE1, ICE2 and ELL. Furthermore, HA-ICE1 was copurified with Myc-EAF1 only in the presence of FLAG-ELL ( Fig. 2b ), indicating that ELL is required for formation of the protein complex containing ICE1, ELL and EAF1. FLAG-ICE2 was copurified with HA-ELL and Myc-EAF1 in the presence of HA-ICE1 ( Fig. 2c ), indicating that ICE1 is required for formation of the protein complex containing ICE1, ICE2, ELL and EAF1. These results raised the possibility that the largest subunit of LEC, ICE1, functions as a core subunit and connects ICE2 and ELL/EAF for the formation of LEC. Considering that EAF1 directly interacts with MED26-NTD [20] , the EAF family protein is thought to function as an adaptor molecule to connect MED26-NTD and LEC ( Fig. 2d ). 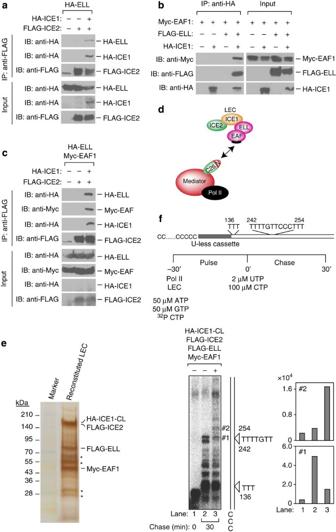Figure 2: Reconstitution of LEC by a baculovirus expression system. (a) ICE2 (NARG2) binds to ELL in the presence of ICE1 (KIAA0947). FLAG-immunopurified complexes from baculovirus-infected Sf9 cells expressing the indicated proteins were analysed by western blot. (b) ICE1 binds to EAF1 in the presence of ELL. HA-immunopurified complexes from baculovirus-infected Sf9 cells expressing the indicated proteins were analysed by western blot. (c) ICE2 binds to ELL/EAF1 in the presence of ICE1. FLAG-immunopurified complexes from baculovirus-infected Sf9 cells expressing the indicated proteins were analysed by western blot. (d) Proposed architecture of the components of LEC and model for MED26-NTD function as a docking site for LEC. MED26-NTD interacts with LEC through direct interaction with EAF. In turn, the MED26 CTD binds to Pol II through Mediator. The binding site for MED26-NTD on EAF is represented by black bars. (e) Silver staining of HA-ICE1-CL/FLAG-ICE2/FLAG-ELL/Myc-EAF1 complex reconstituted by the baculovirus expression system. FLAG-tagged ELL, Myc-tagged EAF1, FLAG-tagged ICE2 and HA-tagged ICE1 C-terminal fragments (CL: 1,191–2,266) were co-expressed in Sf9 insect cells, and the ICE1-CL/ICE2/ELL/EAF1 complex was purified by anti-HA affinity chromatography as described in the Methods section. * indicates heavy and light chains derived from anti-HA antibodies used in affinity purification. (f) ICE1-CL/ICE2/ELL/EAF1 complex enhances transcription elongation by Pol II. Oligo(dC)-tailed template transcription assays were performed as described in the Results and Methods sections. Arrowhead indicates the position of the nascent transcript that is synthesized in the presence of ATP, GTP and CTP and stalled at the T site. Figure 2: Reconstitution of LEC by a baculovirus expression system. ( a ) ICE2 (NARG2) binds to ELL in the presence of ICE1 (KIAA0947). FLAG-immunopurified complexes from baculovirus-infected Sf9 cells expressing the indicated proteins were analysed by western blot. ( b ) ICE1 binds to EAF1 in the presence of ELL. HA-immunopurified complexes from baculovirus-infected Sf9 cells expressing the indicated proteins were analysed by western blot. ( c ) ICE2 binds to ELL/EAF1 in the presence of ICE1. FLAG-immunopurified complexes from baculovirus-infected Sf9 cells expressing the indicated proteins were analysed by western blot. ( d ) Proposed architecture of the components of LEC and model for MED26-NTD function as a docking site for LEC. MED26-NTD interacts with LEC through direct interaction with EAF. In turn, the MED26 CTD binds to Pol II through Mediator. The binding site for MED26-NTD on EAF is represented by black bars. ( e ) Silver staining of HA-ICE1-CL/FLAG-ICE2/FLAG-ELL/Myc-EAF1 complex reconstituted by the baculovirus expression system. FLAG-tagged ELL, Myc-tagged EAF1, FLAG-tagged ICE2 and HA-tagged ICE1 C-terminal fragments (CL: 1,191–2,266) were co-expressed in Sf9 insect cells, and the ICE1-CL/ICE2/ELL/EAF1 complex was purified by anti-HA affinity chromatography as described in the Methods section. * indicates heavy and light chains derived from anti-HA antibodies used in affinity purification. ( f ) ICE1-CL/ICE2/ELL/EAF1 complex enhances transcription elongation by Pol II. Oligo(dC)-tailed template transcription assays were performed as described in the Results and Methods sections. Arrowhead indicates the position of the nascent transcript that is synthesized in the presence of ATP, GTP and CTP and stalled at the T site. Full size image To clarify the region of ICE1 critical for the direct interaction with ICE2 and ELL, we generated recombinant proteins of two truncate mutants of ICE1. The C-terminal fragment of ICE1 (C-terminal long (CL): 1,191–2,266) bound to ICE2, but the N-terminal fragment of ICE1 (N-terminal long (NL): 1–1,190) did not ( Supplementary Fig. 1a ). On the other hand, both NL and CL of ICE1 bound to ELL ( Supplementary Fig. 1b ). These results indicate that the C-terminal fragment of ICE1 is sufficient for the formation of LEC. Consistent with these results, FLAG-ICE1-CL purified from 293FRT cells stably expressing FLAG-ICE1-CL was copurified with LEC components ELL and EAF1 and with Mediator subunits MED26 and MED1 ( Supplementary Fig. 1c ). Taken together, these findings suggest that the C-terminal fragment of ICE1 (CL: 1,191–2,266) functions as a core region for the formation of LEC. LEC enhances transcription elongation of Pol II in vitro To determine whether LEC activates transcription elongation activity of Pol II, we reconstituted LEC using a baculovirus expression system. Since it was difficult to express a sufficient amount of full-length ICE1 (full length (FL): 1–2,266) for transcription assays, we used the C-terminal fragment of ICE1 (CL: 1,191–2,266). HA-ICE1-CL/FLAG-ICE2/FLAG-ELL/Myc-EAF1 complex was reconstituted by a baculovirus expression system ( Fig. 2e ), and in vitro transcription elongation assays were performed to determine whether the complex stimulates Pol II transcription elongation. We used a linearized plasmid with a single-stranded 3′ oligo(dC) tail on its template strand. Although purified Pol II is unable to bind to double-stranded DNA and initiate transcription without assistance from the general transcription factors, it binds to the single-stranded oligo(dC) tail and initiates transcription specifically at the junction between the single- and double-stranded regions of the template. In the template, the first nontemplate strand (dT) residue is 136 nt downstream of the oligo(dC) tail, and the next run of (dT) residues is located ≈240 to ≈250 residues from the oligo(dC) tail ( Fig. 2f , upper panel). When transcription was initiated by the addition of purified Pol II, 50 μM ATP, 50 μM GTP, 2 μM CTP and 10 μCi [α- 32 P]CTP ( Fig. 2f , upper panel), labelled 135-nt transcripts paused immediately before the first template T residue accumulated ( Fig. 2f , lower left panel, lane 1). After 30 min, reactions were chased with 100 μM CTP and 2 μM UTP in the absence or presence of HA-ICE1-CL/FLAG-ICE2/FLAG-ELL/Myc-EAF1 complex as indicated ( Fig. 2f , lower left panel, lanes 2 and 3). When the complex was added with chase nucleotides, the fraction of Pol II that was able to read through the major pause site synthesized longer transcripts ( Fig. 2f , lane 3). Quantification of the major paused transcript (#1) and the longer transcript (#2) supports our idea that reconstituted LEC helps Pol II to read through the major pause site and synthesize the longer transcript ( Fig. 2f , lower right panel). These results showed that reconstituted LEC enhances transcription elongation of Pol II in vitro . MED26 is required for the occupancy of LEC at snRNA genes To identify the genes in which LEC is present, we performed chromatin immunoprecipitation-sequence (ChIP-seq) analysis of the LEC component ICE1. By plotting the occupancy of ICE1 at the transcription start sites (TSSs), we identified 117 genes. Forty-six of these genes were snRNA or snoRNA genes ( Supplementary Data 1 ). These data are consistent with the results of previous studies showing that LEC plays a role in transcription of Pol II-transcribed snRNA genes [12] , [13] . To determine whether MED26 plays a role in recruitment of LEC, we performed ChIP-seq analysis of ICE1 using chromatin from HEK293T cells that had been transfected with control small interfering RNA (siRNA) or MED26 siRNA. By plotting the occupancy of ICE1 at known TSS in cells treated with control siRNA, a subset of snRNA and snoRNA genes was shown to be occupied by ICE1 ( Fig. 3a–d ; Supplementary Fig. 2a–c ; Supplementary Data 2 ). On siRNA-mediated depletion of MED26, almost all of the ChIP peaks of ICE1 at snRNA genes were decreased ( Fig. 3a–d ; Supplementary Fig. 2a–c ), indicating that MED26 is critical for the occupancy of ICE1 at a subset of snRNA genes. In control experiments, we confirmed that MED26 depletion had no significant effect on the expression of Mediator subunit MED1, any of LEC components tested and Pol II subunit Rpb1 ( Fig. 3e ). Next we performed ChIP-quantitative PCR (qPCR) of ICE1 using probes for a subset of snRNA genes and CELF3 gene in which peaks of ICE1 were detected in ChIP-seq analysis ( Supplementary Data 1 and 2 ) and using the Pol III-transcribed U6 gene as a negative control. Consistent with the results of ChIP-seq analysis of ICE1, ICE1 was significantly occupied at the U1-1 , U4-1 , U5A and U5B snRNA genes and CELF3 gene compared with the U6 snRNA gene ( Fig. 3f ). MED26 knockdown decreased the occupancy of ICE1 significantly at U1-1 , U4-1 , U5A and U5B snRNA genes but not at the CELF3 gene ( Fig. 3f ), indicating that depletion of MED26 specifically decreased the occupancy of ICE1 at a subset of snRNA genes. MED26 knockdown decreased the occupancy of other LEC components, ELL and EAF2, at U1 , U4-1 , U5A and U5B snRNA genes ( Fig. 3f ). These data show that MED26 is required for the occupancy of LEC at a subset of snRNA genes. 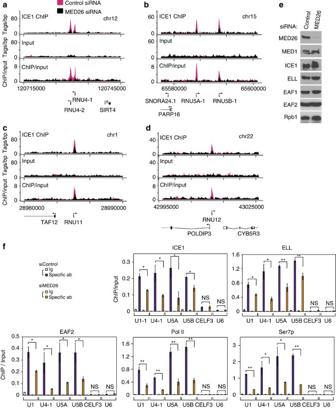Figure 3: MED26 is needed for the occupancy of LEC at a subset ofsnRNAgenes. (a–d) Depletion of MED26 decreases the occupancy of ICE1 (KIAA0947) at a subset of Pol II-transcribedsnRNAgenes. ChIP-seq analysis was performed using triplicate ChIP samples. Genome browser track examples showing the effect of MED26 depletion on ICE1 occupancy at a subset ofsnRNAgenes includingRNU4-1andRNU4-2(a),RNU5AandRNU5B(b),RNU11(c) andRNU12(d) were depicted by averaging three of each sequence read from triplicate ChIPs. (e) Western blot showing Mediator, Pol II and LEC components in HEK293T cells treated with non-targeting siRNA or MED26 siRNA#1. (f) Knockdown of MED26 decreases the occupancy of ICE1, ELL, EAF2 and total and Ser7-phosphorylated Pol II at a subset ofsnRNAgenes.Ctvalues of each ChIP were normalized to that of input. Each value is the average of three independent experiments, and error bars show s.d. ThePvalues for the indicated comparisons were determined by Student’st-test (*P<0.05; **P<0.01). Figure 3: MED26 is needed for the occupancy of LEC at a subset of snRNA genes. ( a – d ) Depletion of MED26 decreases the occupancy of ICE1 (KIAA0947) at a subset of Pol II-transcribed snRNA genes. ChIP-seq analysis was performed using triplicate ChIP samples. Genome browser track examples showing the effect of MED26 depletion on ICE1 occupancy at a subset of snRNA genes including RNU4-1 and RNU4-2 ( a ), RNU5A and RNU5B ( b ), RNU11 ( c ) and RNU12 ( d ) were depicted by averaging three of each sequence read from triplicate ChIPs. ( e ) Western blot showing Mediator, Pol II and LEC components in HEK293T cells treated with non-targeting siRNA or MED26 siRNA#1. ( f ) Knockdown of MED26 decreases the occupancy of ICE1, ELL, EAF2 and total and Ser7-phosphorylated Pol II at a subset of snRNA genes. C t values of each ChIP were normalized to that of input. Each value is the average of three independent experiments, and error bars show s.d. The P values for the indicated comparisons were determined by Student’s t -test (* P <0.05; ** P <0.01). Full size image Transcription of snRNA genes by Pol II is associated with Ser7 phosphorylation of Pol II CTD [16] . Depletion of MED26 decreased the occupancy of total Pol II (Rpb1), accompanied by a decrease in the occupancy of Ser7-phosphorylated Pol II at snRNA genes ( Fig. 3f ). These results suggest that MED26 contributes to Pol II recruitment and/or Ser7 phosphorylation of Pol II CTD at snRNA genes. MED26-containing Mediator is present at snRNA genes To test whether Mediator was present at snRNA genes, we performed ChIP of Mediator subunits, MED26, MED23 and MED1, followed by qPCR using probes for the c-Myc gene and snRNA genes including U1-1 , U4-1 , U4-2 , U5A , U5B and U6 ( Fig. 4a ). Consistent with the results of a previous study showing that MED26 plays a role in recruitment of SEC to the c-Myc gene, MED26, MED23 and MED1 were present at the promoter region of the c-Myc gene ( Fig. 4b ). Significantly larger amounts of MED26, MED23 and MED1 were present at snRNA genes including U1-1 , U4-1 , U4-2 , U5A and U5B than those at the upstream or downstream regions of the respective genes and U6 snRNA gene ( Fig. 4b ). These results showed that Mediator was present at a subset of snRNA genes. 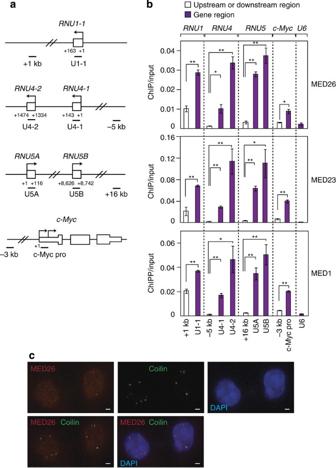Figure 4: MED26-containing Mediator is present at a subset ofsnRNAgenes. (a) Diagram of the genes and primer locations used for ChIP. (b) Occupancy of Mediator subunits MED26, MED23 and MED1 at a subset ofsnRNAgenes includingRNU1,RNU4,RNU5andU6, andc-Mycgenes.Ctvalues of each ChIP were normalized to that of input. Data points are the average of three independent experiments, and error bars show s.d. ThePvalues for the indicated comparisons were determined by Student’st-test (*P<0.05; **P<0.01). (c) Co-localization of MED26 (red) with coilin (green) in Cajal bodies. HeLa cells were fixed by methanol and stained with anti-MED26 and anti-coilin antibodies. Scale bars, 2 μm. Figure 4: MED26-containing Mediator is present at a subset of snRNA genes. ( a ) Diagram of the genes and primer locations used for ChIP. ( b ) Occupancy of Mediator subunits MED26, MED23 and MED1 at a subset of snRNA genes including RNU1 , RNU4 , RNU5 and U6 , and c-Myc genes. C t values of each ChIP were normalized to that of input. Data points are the average of three independent experiments, and error bars show s.d. The P values for the indicated comparisons were determined by Student’s t -test (* P <0.05; ** P <0.01). ( c ) Co-localization of MED26 (red) with coilin (green) in Cajal bodies. HeLa cells were fixed by methanol and stained with anti-MED26 and anti-coilin antibodies. Scale bars, 2 μm. Full size image It was previously shown that LEC was co-localized at Cajal bodies [13] . Cajal bodies were shown to be the sites for not only pre-mRNA splicing, but also transcription of snRNA genes [32] . We therefore investigated whether MED26 was also co-localized with coilin, which is widely used as a molecular marker of Cajal bodies. We performed immunostaining of ICE1 and MED26 using HeLa cells. ICE1 was co-localized with coilin in Cajal bodies ( Supplementary Fig. 3 ). MED26 was stained diffusely in the nucleus and partly formed nuclear dots in which coilin was co-localized ( Fig. 4c ). These results indicate that MED26-containing Mediator is co-localized with coilin at Cajal bodies and are consistent with our idea that MED26 has a role in transcription of snRNA genes. MED26 is required for the expression of snRNA genes To test whether depletion of MED26 affects the expression of snRNA genes, total RNAs were extracted from HEK293T cells that had been transfected with control siRNA or one of three different MED26 siRNAs ( Supplementary Fig. 4a ). Reverse transcription–qPCR (RT–qPCR) analysis revealed that the expression of a subset of snRNA and snoRNA genes, including U1 , U2 , U4-1 , U4-2 , U5A , U5B , U11 and snord118 , was decreased following transfection of all three MED26 siRNAs, but the expression of U6 snRNA genes was not changed by depletion of MED26 ( Fig. 5a ). These findings show that MED26 is required for the expression of snRNA genes. 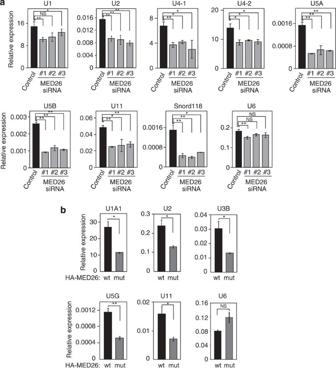Figure 5: MED26 is required for the expression of Pol II-transcribedsnRNAandsmall nucleolar RNA (snoRNA)genes. (a) MED26 depletion in cells decreases the expression of a subset of Pol II-transcribedsnRNAandsnoRNAgenes. HEK293T cells were transfected with non-targeting siRNA as a control and each of three different siRNAs (#1, #2 and #3) targeting MED26. Total RNAs were extracted from cells and the expression of indicated genes was measured by real-time qPCR.Ctvalues were normalized to GAPDH. Data points are the average of three independent experiments, and error bars show s.d. ThePvalues for the indicated comparisons were determined by Student’st-test (*P<0.04; **P<0.008). (b) MED26 wt contributes more to the expression of a subset ofsnRNAgenes than does a MED26 point mutant (mut: R61A, K62A). Total RNAs were extracted from MED26 gene-trapped MEF cells expressing HA-tagged MED26 wt or point mutant (mut), and the expression of the indicated genes was measured by real-time qPCR.Ctvalues were normalized to GAPDH. Data points are the average of three independent experiments, and error bars show s.d. ThePvalues for the indicated comparisons were determined by Student’st-test (*P<0.04; **P<0.008). Figure 5: MED26 is required for the expression of Pol II-transcribed snRNA and small nucleolar RNA (snoRNA) genes. ( a ) MED26 depletion in cells decreases the expression of a subset of Pol II-transcribed snRNA and snoRNA genes. HEK293T cells were transfected with non-targeting siRNA as a control and each of three different siRNAs (#1, #2 and #3) targeting MED26. Total RNAs were extracted from cells and the expression of indicated genes was measured by real-time qPCR. C t values were normalized to GAPDH. Data points are the average of three independent experiments, and error bars show s.d. The P values for the indicated comparisons were determined by Student’s t -test (* P <0.04; ** P <0.008). ( b ) MED26 wt contributes more to the expression of a subset of snRNA genes than does a MED26 point mutant (mut: R61A, K62A). Total RNAs were extracted from MED26 gene-trapped MEF cells expressing HA-tagged MED26 wt or point mutant (mut), and the expression of the indicated genes was measured by real-time qPCR. C t values were normalized to GAPDH. Data points are the average of three independent experiments, and error bars show s.d. The P values for the indicated comparisons were determined by Student’s t -test (* P <0.04; ** P <0.008). Full size image To assess the potential contribution of MED26-NTD to the transcription of snRNA genes, we generated mouse embryonic fibroblast (MEF) cells from day 10.5 homozygous embryos in which a gene trapping construct had been inserted into the first intron of the mouse MED26 gene. Consistent with the results of a recent study showing that MED26 is critical for organismal viability but not for cell survival in Drosophila [33] , MEF cells from MED26 gene trap homozygous embryos were alive and expressed house-keeping protein GAPDH and Mediator subunit MED18 at levels similar to those in MEF cells from wild-type embryos. In contrast, the expression of MED26 in MEF cells was undetectable, unlike that in wild-type embryos ( Supplementary Fig. 4b ). To investigate the contribution of MED26-NTD to snRNA gene expression in cells, MED26 wild type and MED26-R61A, K62A, which did not interact with LEC ( Fig. 1b ), were stably expressed in MEF cells from MED26 gene trap homozygous embryos. We confirmed that MED26-R61A, K62A was expressed at the same level as that of MED26 wild type and that it had no significant effect on the expression of MED1, Rpb1 and heat–shock protein 90 (Hsp90; Supplementary Fig. 4c ). The expression levels of mouse U1A1 , U2 , U3B , U5G and U11 snRNA genes, but not the expression level of the U6 snRNA gene, were significantly higher in MEF cells expressing MED26 wild type than in MEF cells expressing MED26-R61A, K62A ( Fig. 5b ). These results indicate that MED26-NTD contributes to the expression of snRNA genes through the recruitment of LEC. Region of EAF1 necessary for interaction with MED26-NTD Since we previously found that EAF1 directly bound to MED26-NTD [20] , we carried out an experiment to determine the region of human EAF1 responsible for interaction with MED26-NTD. We tested whether recombinant proteins of a series of HA-EAF1 C-terminal deletion mutants bound to FLAG-MED26-NTD ( Fig. 6a ). The full length (FL) of EAF1 bound to MED26-NTD, but the C-terminal deletion mutant N244 did not ( Fig. 6b ), indicating that C-terminal amino-acid residues from 245 to 268 in human EAF1 are required for interaction with MED26-NTD. 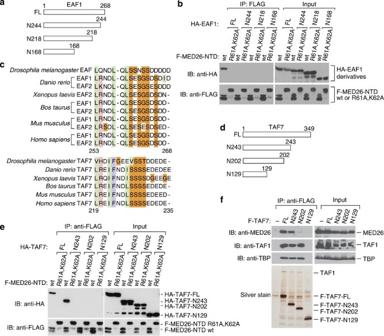Figure 6: Similarity of EAF and TAF7 in amino-acids sequence that is necessary for interaction with MED26-NTD. (a) Schematic representation of deletion mutants of human EAF1. (b) Binding ability of deletion mutants of EAF1 with MED26-NTD. The indicated recombinant proteins were expressed in Sf9 cells. Recombinant proteins of FLAG-tagged MED26-NTD derivatives were immobilized on anti-FLAG M2 agarose and were then incubated with the lysate from Sf9 cells expressing each deletion mutant of HA-tagged EAF1. After washing, bound proteins were eluted and analysed by western blot. F-MED26-NTD R61A, K62A has a larger molecular weight than that of F-MED26-NTD wt since the linker between the N-terminal hexa-histidine tag and FLAG tag of MED26-NTD R61A, K62A is longer than that of MED26-NTD wt. (c) Sequence alignment of EAF and TAF7 in amino-acid sequence that is required for interaction with MED26-NTD. Light green column indicates hydrophobic residues. Pink column indicates basic residues. Light blue column indicates aromatic residues. Orange column indicates neutral residues. The indicated number of amino acids is fromHomo sapiensEAF1 and TAF7, respectively. (d) Schematic representation of deletion mutants of human TAF7. (e) Binding ability of deletion mutants of TAF7 with MED26-NTD. The indicated recombinant proteins were expressed in Sf9 cells. Recombinant proteins of FLAG-tagged MED26-NTD derivatives were immobilized on anti-FLAG M2 agarose and were then incubated with the lysate from Sf9 cells expressing each deletion mutant of HA-tagged TAF7. After washing, bound proteins were eluted and analysed by western blot. F-MED26-NTD R61A, K62A has a larger molecular weight than that of F-MED26-NTD wt since the linker between the N-terminal hexa-histidine tag and FLAG tag of MED26-NTD R61A, K62A is longer than that of MED26-NTD wt. (f) Western blot analysis of FLAG-immunopurified complexes from parental HeLa cells (control) and HeLa cells stably expressing FLAG-tagged TAF7 full length (FL) and C-terminal deletion mutants, N243 (1–243), N202 (1–202) and N129 (1–129). Figure 6: Similarity of EAF and TAF7 in amino-acids sequence that is necessary for interaction with MED26-NTD. ( a ) Schematic representation of deletion mutants of human EAF1. ( b ) Binding ability of deletion mutants of EAF1 with MED26-NTD. The indicated recombinant proteins were expressed in Sf9 cells. Recombinant proteins of FLAG-tagged MED26-NTD derivatives were immobilized on anti-FLAG M2 agarose and were then incubated with the lysate from Sf9 cells expressing each deletion mutant of HA-tagged EAF1. After washing, bound proteins were eluted and analysed by western blot. F-MED26-NTD R61A, K62A has a larger molecular weight than that of F-MED26-NTD wt since the linker between the N-terminal hexa-histidine tag and FLAG tag of MED26-NTD R61A, K62A is longer than that of MED26-NTD wt. ( c ) Sequence alignment of EAF and TAF7 in amino-acid sequence that is required for interaction with MED26-NTD. Light green column indicates hydrophobic residues. Pink column indicates basic residues. Light blue column indicates aromatic residues. Orange column indicates neutral residues. The indicated number of amino acids is from Homo sapiens EAF1 and TAF7, respectively. ( d ) Schematic representation of deletion mutants of human TAF7. ( e ) Binding ability of deletion mutants of TAF7 with MED26-NTD. The indicated recombinant proteins were expressed in Sf9 cells. Recombinant proteins of FLAG-tagged MED26-NTD derivatives were immobilized on anti-FLAG M2 agarose and were then incubated with the lysate from Sf9 cells expressing each deletion mutant of HA-tagged TAF7. After washing, bound proteins were eluted and analysed by western blot. F-MED26-NTD R61A, K62A has a larger molecular weight than that of F-MED26-NTD wt since the linker between the N-terminal hexa-histidine tag and FLAG tag of MED26-NTD R61A, K62A is longer than that of MED26-NTD wt. ( f ) Western blot analysis of FLAG-immunopurified complexes from parental HeLa cells (control) and HeLa cells stably expressing FLAG-tagged TAF7 full length (FL) and C-terminal deletion mutants, N243 (1–243), N202 (1–202) and N129 (1–129). Full size image Comparison of MED26-NTD-binding regions in EAF and TAF7 Since we previously found that EAF and TFIID bind to the overlapping binding site of MED26-NTD and that EAF1 recruitment by Mediator is inhibited by TFIID in vitro [20] , we considered the possibility that a certain TBP-associated factor (TAF) directly interacts with MED26-NTD. First, we investigated which TAFs directly interact with MED26-NTD. We performed in vitro binding assays using bacterially expressed glutathione S-transferase (GST)-MED26 and a pool of 13 kinds of human TAFs (from TAF1 to TAF13) expressed in a baculovirus expression system and tested which TAFs were pulled down by GST-MED26. We found that TAF1 and TAF7 were copurified with GST-MED26 but not with GST alone. To test whether TAF7 directly interacts with MED26-NTD, we performed in vitro binding assays using bacterially expressed FLAG-MED26-NTD and HA-TAF7. TAF7 directly interacted with MED26-NTD but not with MED26-NTD R61A, K62A ( Supplementary Fig. 5a ). In turn, TAF1 bound to MED26-NTD only in the presence of TAF7 ( Supplementary Fig. 5b ), suggesting that TAF1 interacted with MED26-NTD via TAF7 in the first binding assay with pooled TAFs. This result indicates that MED26-NTD interacts with not only free TAF7, but also TAF7 bound to TAF1, raising the possibility that MED26-NTD interacts with TAF7 in the context of TFIID. Since TAF7 is a subunit of TFIID, it is possible that expression of TAF7 as a single subunit results in aggregation and that recombinant protein of TAF7 does not exist as a monomer. To exclude this possibility, we tested whether recombinant HA-TAF7 and FLAG-TAF7 bind to each other. An in vitro binding assay revealed that HA-TAF7 bound to FLAG-MED26-NTD but not to FLAG-TAF7 ( Supplementary Fig. 5c ). Although it is still possible that recombinant TAF7 proteins form a higher-order state and do not bind to each other, our results suggest that recombinant TAF7 exists at least in part as a monomer. Taken together, our results showed that TAF7 directly bound to MED26-NTD. Next we investigated whether TAF7 harbours an amino-acid sequence similar to that of the MED26-NTD-binding region of EAF1. Sequence alignment revealed that the amino-acid sequence from 219 to 235 in human TAF7 is partially similar to the amino-acid sequence from 253 to 268 in human EAF1 ( Fig. 6c ). Notably, both of the regions in TAF7 and EAF are conserved among species ( Fig. 6c ). To determine whether the region of TAF7 is responsible for interaction with MED26-NTD, we generated recombinant proteins of a series of HA-TAF7 C-terminal deletion mutants ( Fig. 6d ) and FLAG-MED26-NTD by a baculovirus expression system and tested whether these mutants bind to MED26-NTD. FL and N243 (1–243) of TAF7 bound to MED26-NTD, but N202 (1–202) and N129 (1–129) did not ( Fig. 6e ), demonstrating that the region from 203 to 243 is required for interaction with MED26-NTD. We next tested whether the same region of TAF7 is required for interaction with MED26 in cells. FLAG-TAF7 FL and a series of C-terminal deletion mutants were purified from HeLa S3 cells stably expressing each of TAF7 FL and deletion mutants. FLAG-FL and N243 were copurified with MED26, but N202 and N129 were not ( Fig. 6f ), demonstrating that the region from 203 to 243 is required for interaction with MED26 in cells. Consistent with the results of previous studies showing that the amino-acid sequence from 139 to 249 of TAF7 contributes to the binding site for TAF1 (refs 34 , 35 , 36 ), FLAG-TAF7 FL, N243 and N202 were copurified with TFIID components TAF1 and TBP, but N129 was not ( Fig. 6f ). These findings indicate that the region from 203 to 243 of TAF7 is dispensable for interaction with TAF1 or TFIID. Our results indicate that the distinct region of TAF7 contributes to interaction with MED26 and its incorporation into TFIID. Point mutations of TAF7 and EAF1 block binding to MED26 We generated point mutants of EAF1 and TAF7, which lose interaction with MED26-NTD ( Fig. 7a ). Mutations of S262, G263, S264 and D265 to A interfered with the interaction of EAF1 and MED26-NTD ( Fig. 7b ). Similarly, mutations of S229, S230, E231 and D232 to A interfered with the interaction of TAF7 and MED26-NTD ( Fig. 7c ). Consistent with the fact that the region of TAF7 is not well conserved in TAF7L ( Fig. 7a ), TAF7L did not bind to MED26-NTD ( Fig. 7d ). To test whether the region of TAF7 is critical for interaction with MED26 in cells, we generated HeLa cells stably expressing FLAG-TAF7 wild type and point mutant (S229A, S230A, E231A, D232A) and purified TFIID ( Fig. 7e ). Consistent with our results showing that the region of TAF7 is dispensable for interaction with TFIID ( Fig. 6f ), both the wild type and point mutant copurified with similar levels of TFIID components TAF1 and TBP ( Fig. 7f ). In contrast, the wild type of TAF7 copurified with MED26 and MED1, but the point mutant did not ( Fig. 7f ), demonstrating that the region of TAF7 is required for interaction with MED26-containing Mediator. These findings indicate the possibility that TAF7 in the context of TFIID and/or free TAF7 interacts with MED26-containing Mediator. 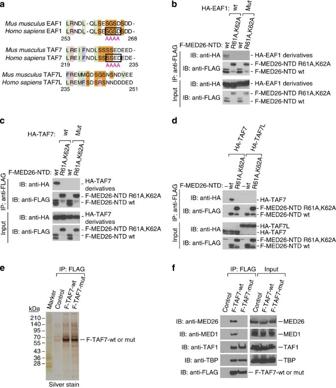Figure 7: Identification of TAF7 and EAF1 mutations that interfere with MED26-NTD binding. (a) Sequence alignment of EAF1, TAF7 and TAF7L in amino-acid sequence that is required for interaction with MED26-NTD. Light green indicates hydrophobic residues. Pink column indicates basic residues. Light blue column indicates aromatic residues. Orange column indicates neutral residues. The residues that are substituted for alanine to generate mutants of EAF1 and TAF7 are surrounded by square. The indicated number of amino acids is from human EAF1 and TAF7, respectively. (b) Substitution of S262, G263, S264 and D265 to A interferes with human EAF1 interaction with MED26-NTD. Recombinant proteins of wt or point mutant (R61A, K62A) of FLAG-tagged MED26-NTD were immobilized on anti-FLAG M2 agarose. The M2 agarose complex was incubated with recombinant proteins of HA-tagged EAF1 wt or point mutant (mut). After washing, bound proteins were eluted and analysed by western blot. (c) Substitution of S229, S230, E231 and D232 to A interferes with human TAF7 interaction with MED26-NTD. Recombinant proteins of wt or point mutant (R61A, K62A) of FLAG-tagged MED26-NTD were immobilized on anti-FLAG M2 agarose. The M2 agarose complex was incubated with recombinant proteins of HA-tagged TAF7 wt or point mutant (mut). After washing, bound proteins were eluted and analysed by western blot. (d) TAF7L does not bind to MED26-NTD. Recombinant proteins of wt or point mutant (R61A, K62A) of FLAG-tagged MED26-NTD were immobilized on anti-FLAG M2 agarose. The M2 agarose complex was incubated with recombinant proteins of HA-tagged human TAF7 or HA-tagged mouse TAF7L. After washing, bound proteins were eluted and analysed by western blot. (e) Silver staining of TFIID purified from HeLa cells stably expressing FLAG-tagged TAF7 wt and point mutant (mut) by anti-FLAG affinity chromatography. (f) Western blot for FLAG-immunopurified complexes from parental HeLa cells (control) and HeLa cells stably expressing FLAG-tagged TAF7 wt and point mutant (mut). Figure 7: Identification of TAF7 and EAF1 mutations that interfere with MED26-NTD binding. ( a ) Sequence alignment of EAF1, TAF7 and TAF7L in amino-acid sequence that is required for interaction with MED26-NTD. Light green indicates hydrophobic residues. Pink column indicates basic residues. Light blue column indicates aromatic residues. Orange column indicates neutral residues. The residues that are substituted for alanine to generate mutants of EAF1 and TAF7 are surrounded by square. The indicated number of amino acids is from human EAF1 and TAF7, respectively. ( b ) Substitution of S262, G263, S264 and D265 to A interferes with human EAF1 interaction with MED26-NTD. Recombinant proteins of wt or point mutant (R61A, K62A) of FLAG-tagged MED26-NTD were immobilized on anti-FLAG M2 agarose. The M2 agarose complex was incubated with recombinant proteins of HA-tagged EAF1 wt or point mutant (mut). After washing, bound proteins were eluted and analysed by western blot. ( c ) Substitution of S229, S230, E231 and D232 to A interferes with human TAF7 interaction with MED26-NTD. Recombinant proteins of wt or point mutant (R61A, K62A) of FLAG-tagged MED26-NTD were immobilized on anti-FLAG M2 agarose. The M2 agarose complex was incubated with recombinant proteins of HA-tagged TAF7 wt or point mutant (mut). After washing, bound proteins were eluted and analysed by western blot. ( d ) TAF7L does not bind to MED26-NTD. Recombinant proteins of wt or point mutant (R61A, K62A) of FLAG-tagged MED26-NTD were immobilized on anti-FLAG M2 agarose. The M2 agarose complex was incubated with recombinant proteins of HA-tagged human TAF7 or HA-tagged mouse TAF7L. After washing, bound proteins were eluted and analysed by western blot. ( e ) Silver staining of TFIID purified from HeLa cells stably expressing FLAG-tagged TAF7 wt and point mutant (mut) by anti-FLAG affinity chromatography. ( f ) Western blot for FLAG-immunopurified complexes from parental HeLa cells (control) and HeLa cells stably expressing FLAG-tagged TAF7 wt and point mutant (mut). Full size image TAF7 is present at snRNA genes To test whether TAF7 is also present at snRNA genes, we compared the peaks of ICE1 (KIAA0947) ChIP-seq and TAF7 ChIP-seq. We identified 2,912 TAF7-bound genes by TSS analysis ( Fig. 8a ; Supplementary Data 3 ). Forty-two genes out of the 117 ICE1-bound genes overlapped with TAF7-co-occupied genes. Notably, most of the 42 genes were snRNA or snoRNA genes ( Fig. 8a ; Supplementary Data 4 ), indicating that TAF7 plays a role in regulating the transcription of snRNA genes. TAF7 was co-localized with ICE1 at a subset of snRNA genes ( Fig. 8b–e ; Supplementary Fig. 6a–c ). ChIP-qPCR analysis also demonstrated that TAF7 was present at a subset of snRNA genes ( Fig. 8f ). 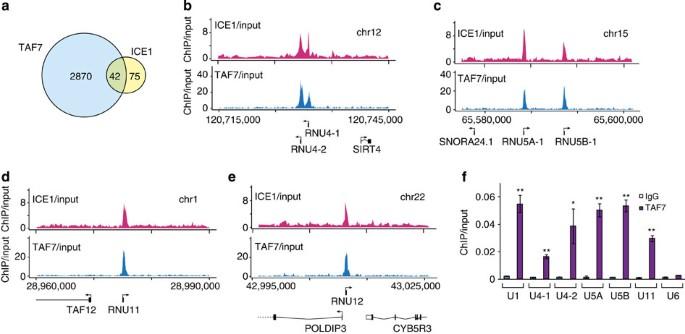Figure 8: TAF7 is present at a subset ofsnRNAgenes. (a) Venn diagram showing the overlap of TAF7- and ICE1 (KIAA0947)-occupied genes. (b–e) TAF7 and ICE1 are present at a subset ofsnRNAgenes. Comparison of the genome browser tracks showing ICE1 and TAF7 ChIP-seq analysis. ChIP-seq tracks of ICE1 (pink) are fromFig. 3a–d. (f) Occupancy of TAF7 at a subset ofsnRNAgenes.Ctvalues of each ChIP were normalized to that of input. Each value is the average of three independent experiments, and error bars show s.d. ThePvalues for the indicated comparisons were determined by Student’st-test (*P<0.05; **P<0.01). Figure 8: TAF7 is present at a subset of snRNA genes. ( a ) Venn diagram showing the overlap of TAF7- and ICE1 (KIAA0947)-occupied genes. ( b – e ) TAF7 and ICE1 are present at a subset of snRNA genes. Comparison of the genome browser tracks showing ICE1 and TAF7 ChIP-seq analysis. ChIP-seq tracks of ICE1 (pink) are from Fig. 3a–d . ( f ) Occupancy of TAF7 at a subset of snRNA genes. C t values of each ChIP were normalized to that of input. Each value is the average of three independent experiments, and error bars show s.d. The P values for the indicated comparisons were determined by Student’s t -test (* P <0.05; ** P <0.01). Full size image Knockdown of TAF7 increases LEC recruitment to snRNA genes Next we tested how depletion of TAF7 in cells affects the expression of snRNA genes. We performed qRT–PCR to analyse snRNA gene expression in HEK293T cells in which TAF7 had been depleted by transient transfection of siRNA ( Fig. 9a ). Knockdown of TAF7 mildly increased the expression of snRNA genes ( Fig. 9b ). 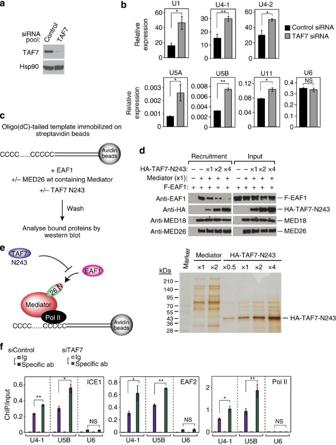Figure 9: Depletion of TAF7 in cells increases the occupancy of LEC at Pol II-transcribedsnRNAgenes. (a) Western blot showing TAF7 and Hsp90 at 48 h after transient transfection of non-targeting (control) siRNA pool or siRNA pool targeting TAF7. (b) Effect of TAF7 depletion on transcript levels of Pol II-transcribedsnRNAgenes detected by RT–qPCR performed with total RNA from cells transfected with siRNAs.Ctvalues were normalized to GAPDH. Data points are the average of three independent experiments, and error bars show s.d. ThePvalues for the indicated comparisons were determined by Student’st-test (*P<0.05; **P<0.01). (c) Schematic representation of immobilized oligo(dC)-tailed template assay. Templates immobilized on streptavidin beads were incubated with purified recombinant protein EAF1 in the presence or absence of Mediator and/or TAF7 N243. After washing, bead-bound proteins were detected by western blot. (d) TAF7 interferes with EAF1 recruitment by Mediatorin vitro. Upper panel shows immobilized oligo(dC)-tailed template assays. Assays were performed with an oligo(dC)-tailed template, EAF1, and Mediator in the presence or absence of TAF7 N243. Lower panel shows silver staining of Mediator and HA-tagged TAF7 N243 used in the assay. Mediator (× 1) and HA-TAF7 N243 (× 1) contain 1 pmol of the each protein or protein complex. (e) Model of immobilized oligo(dC)-tailed template assay. TAF7 N243 inhibits EAF1 recruitment to the oligo(dC)-tailed template by MED26-containing Mediator. (f) Depletion of TAF7 increased the occupancy of ICE1 (KIAA0947), EAF2 and total Pol II atU4-1andU5BsnRNA genes.Ctvalues of each ChIP were normalized to that of input. Data points are the average of three independent experiments, and error bars show s.d. ThePvalues for the indicated comparisons were determined by Student’st-test (*P<0.05; **P<0.01). Figure 9: Depletion of TAF7 in cells increases the occupancy of LEC at Pol II-transcribed snRNA genes. ( a ) Western blot showing TAF7 and Hsp90 at 48 h after transient transfection of non-targeting (control) siRNA pool or siRNA pool targeting TAF7. ( b ) Effect of TAF7 depletion on transcript levels of Pol II-transcribed snRNA genes detected by RT–qPCR performed with total RNA from cells transfected with siRNAs. C t values were normalized to GAPDH. Data points are the average of three independent experiments, and error bars show s.d. The P values for the indicated comparisons were determined by Student’s t -test (* P <0.05; ** P <0.01). ( c ) Schematic representation of immobilized oligo(dC)-tailed template assay. Templates immobilized on streptavidin beads were incubated with purified recombinant protein EAF1 in the presence or absence of Mediator and/or TAF7 N243. After washing, bead-bound proteins were detected by western blot. ( d ) TAF7 interferes with EAF1 recruitment by Mediator in vitro . Upper panel shows immobilized oligo(dC)-tailed template assays. Assays were performed with an oligo(dC)-tailed template, EAF1, and Mediator in the presence or absence of TAF7 N243. Lower panel shows silver staining of Mediator and HA-tagged TAF7 N243 used in the assay. Mediator (× 1) and HA-TAF7 N243 (× 1) contain 1 pmol of the each protein or protein complex. ( e ) Model of immobilized oligo(dC)-tailed template assay. TAF7 N243 inhibits EAF1 recruitment to the oligo(dC)-tailed template by MED26-containing Mediator. ( f ) Depletion of TAF7 increased the occupancy of ICE1 (KIAA0947), EAF2 and total Pol II at U4-1 and U5B snRNA genes. C t values of each ChIP were normalized to that of input. Data points are the average of three independent experiments, and error bars show s.d. The P values for the indicated comparisons were determined by Student’s t -test (* P <0.05; ** P <0.01). Full size image Since partially similar amino-acid sequences of TAF7 and EAF1 contribute to interaction with MED26-NTD, we considered the possibility that EAF1 and TAF7 bind to MED26-NTD in a mutually exclusive manner and that TAF7 inhibits EAF1 recruitment by Mediator. To test this possibility, we performed an immobilized template recruitment assay using an oligo(dC)-tailed template immobilized on streptavidin beads ( Fig. 9c ). Since sub-stoichiometric Pol II is copurified with MED26-containing Mediator and Pol II binds to the single-stranded oligo(dC) tail, MED26-containing Mediator binds to the oligo(dC)-tailed template via Pol II without any assistance of DNA-binding transcription activators. Using the template, we tested whether MED26-containing Mediator recruits EAF1 to the template ( Supplementary Fig. 7a ). MED26-containing Mediator recruited EAF1 to the template, but MED26 mut (R61A, K62A)-containing Mediator did not ( Supplementary Fig. 7b ). Next we performed immobilized template assays in the presence and absence of MED26-containing Mediator and recombinant proteins of EAF1 and N243 of TAF7 and tested whether TAF7 inhibits EAF1 recruitment by MED26-containing Mediator ( Fig. 9c ). TAF7 N243 inhibited EAF1 recruitment by Mediator in a dose-dependent manner ( Fig. 9d ), indicating that TAF7 N243 binds to MED26-NTD and blocks EAF1 recruitment ( Fig. 9e ). Next we tested whether TAF7 knockdown increases the occupancy of LEC at snRNA genes in cells. TAF7 depletion moderately increased the occupancy of the components of LEC including ICE1, EAF2 and Pol II at U4-1 and U5B snRNA genes ( Fig. 9f ), but it did not affect the occupancy of MED1 and MED26 at snRNA genes ( Supplementary Fig. 7c ). These findings suggest that TAF7 plays a role in repression of the transcription of a subset of snRNA genes through interfering with the recruitment of LEC to a subset of Pol II-transcribed snRNA genes. In this report, we present evidence that the human Mediator subunit MED26 contributes to the recruitment of LEC to a subset of Pol II-transcribed snRNA genes. MED26 depletion in cells decreased the expression of snRNA genes and the occupancy of LEC components at the genes. Molecular genetic approaches using MEF cells from MED26 gene trap homozygous embryos have revealed that wild-type MED26 contributes more to the expression of snRNA genes than does a MED26 point mutant that does not interact with LEC. Our results indicate that Mediator plays a crucial role in the transcription of snRNA genes through recruitment of LEC. Our results are also consistent with evidence that a meta-coactivator complex containing Mediator and Ada-Two-A-containing histone acetyltransferase play a role in transcription of a subset of snRNA genes in mouse embryonic stem (ES) cells [37] . In a recent study, LEC was copurified with TFIIH [38] . Notably, knockdown of ELL as well as components of TFIIH reduced global RNA synthesis after ultraviolet irradiation, indicating that ELL plays a role in the restart of transcription after transcription-coupled DNA repair (TCR) [38] . This evidence indicates the possibility that LEC plays a role in TCR in snRNA gene transcription. Our results indicate that Mediator can function as a key coordinator by orchestrating multiple coregulator complexes and regulate the expression of a subset of snRNA genes possibly through activating transcription elongation and/or reactivating paused Pol II after TCR. This study and our previous research suggest that MED26-NTD contributes to the recruitment of SEC and LEC to Pol II-transcribed protein-coding genes and snRNA genes, respectively, through direct interaction with EAF [20] . However, the hypothesis does not completely explain the mechanisms by which target genes of SEC and LEC are determined, because EAF is a shared component of both SEC and LEC. It is conceivable that other factors also contribute to the determination of target genes of SEC or LEC. A recent study showed that depletion of ICE1 also decreased the occupancy of other LEC components at snRNA genes, indicating that ICE1 functions as a scaffold protein for LEC and contributes to the recruitment of LEC to the promoter [13] . It has also been reported that the minor difference in U1 and U6 promoters results in a slight conformational change of snRNA-activating protein complex (SNAPc) and could determine the Pol II and Pol III specificities of the U1 and U6 promoters [39] . The results of those studies and our study raise the possibility that a combination of MED26, ICE1, SNAPc and other factors contributes to the LEC recruitment to snRNA genes. It has been shown that LEC contains additional components, UPSL1 and ZC3H8 (refs 12 , 13 , 40 ). In our mass spectrometric analysis of MED26-NTD-interacting proteins, we identified ICE1 (KIAA0947), ICE2 (NARG2), ELL and EAF, but not UPSL1 and ZC3H8, as interacting proteins [20] , suggesting that a form of LEC composed of ICE1, ICE2, ELL and EAF is recruited to the promoters by Mediator. We found that EAF and TAF7 harbour a partially similar amino-acid sequence that is necessary for direct interaction with MED26-NTD. We presented evidence that TAF7 is present at a subset of snRNA genes. We found that TAF7 blocks EAF1 recruitment by Mediator in vitro and that depletion of TAF7 in cells increased the occupancy of LEC and Pol II at a subset of snRNA genes, resulting in an increase in the expression of the genes. Our results are consistent with the results of previous studies showing that TAF7 has a role in repression of the transcription of a subset of genes [30] , [41] . TAF7 was shown to inhibit TAF1 acetyltransferase activity, which is necessary for transcription initiation. The release of TAF7 from TFIID allows transcription initiation, indicating that TAF7 functions as a checkpoint factor of transcription initiation and represses TFIID-dependent transcription initiation by preventing premature transcription initiation [35] . It has also been shown that depletion of Mediator subunits decreases transcription of the metallothionein A gene and that depletion of both TAFs and Mediator subunits restores the transcription [42] , suggesting that transcription of the gene is regulated by the balance of TFIID and Mediator. This report is consistent with our results suggesting that the transcription of a subset of snRNA genes is regulated by the balance of TAF7-containing TFIID and MED26-containing Mediator. TBP and some of the TAFs have been shown to be involved in the transcription of snRNA genes [43] , [44] . Our results raise the possibility that TAF7 in the context of TFIID is involved in snRNA gene transcription; however, further experiments are needed to address the precise composition of the form of TBP-TAFs in snRNA gene transcription. The results of our study raise the possibility that TAF7 occludes the MED26-NTD and interferes with the recruitment of LEC in the step of initiation or the very early step of elongation to prevent premature transcription elongation. After TAF7 is released from MED26-NTD on an appropriate signal, LEC can be recruited to the genes through direct interaction of EAF and MED26-NTD to facilitate the transition from initiation to elongation in transcription of a subset of snRNA genes ( Fig. 10 ). 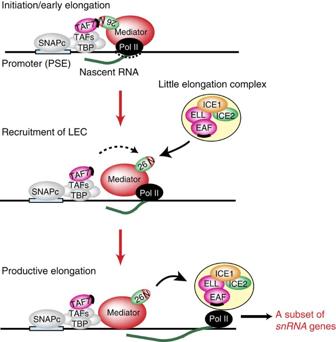Figure 10: Model for MED26 and TAF7 function duringsnRNAgene transcription. In the initiation or early elongation stage, TAF7 interacts with MED26-NTD and blocks LEC recruitment by MED26. In the transition from initiation to elongation, MED26-NTD is released from TAF7 and LEC is recruited to a subset ofsnRNAgenes. After LEC is recruited by MED26, MED26 hands LEC to Pol II, and thereby LEC activates productive elongation of Pol II. Binding sites for the MED26-NTD on TAF7 and EAF family members are represented by black bars. N, MED26-NTD. Figure 10: Model for MED26 and TAF7 function during snRNA gene transcription. In the initiation or early elongation stage, TAF7 interacts with MED26-NTD and blocks LEC recruitment by MED26. In the transition from initiation to elongation, MED26-NTD is released from TAF7 and LEC is recruited to a subset of snRNA genes. After LEC is recruited by MED26, MED26 hands LEC to Pol II, and thereby LEC activates productive elongation of Pol II. Binding sites for the MED26-NTD on TAF7 and EAF family members are represented by black bars. N, MED26-NTD. Full size image Cell culture Human embryonic kidney 293T cells, HeLa cells, HeLa S3 cells and their derivatives, and Flp-In 293 cells (Invitrogen, Carlsbad, CA) and their derivatives were cultured under an atmosphere of 5% CO 2 at 37 °C in DMEM (Sigma-Aldrich Corp., St Louis, MO) supplemented with 10% (v/v) fetal bovine serum (Invitrogen), 55 μM β-mercaptoethanol (Gibco, Grand Island, NY), 2 mM L -glutamine, penicillin (10 U ml −1 ) and streptomycin (0.1 mg ml −1 ). Generation of a HeLa S3 cell line stably expressing FLAG-tagged MED26 wild type, CS (421–600) and R61A, K62A and Flp-In 293 cells stably expressing FLAG-tagged ICE2 and ICE1-CL (1,191–2,266) were described previously [20] . Production of recombinant proteins N-terminally 6 × His- and FLAG-tagged MED26-NTD (residues 1–113), MED26-NTD R61A, K62A and N-terminally 6 × His- and HA-tagged TAF7 were expressed in BL21 (DE3) CodonPlus Escherichia coli (Stratagene, La Jolla, CA) and then purified by using ProBond metal affinity beads (Invitrogen). For production of recombinant proteins in Sf9 cells, epitope-tagged ELL, EAF1 and MED26 were subcloned into pBacPAK8 expressed using the BacPAK system (Clontech Laboratories, Mountain View, CA). Full length, deletion mutants or point mutants of ICE1 (KIAA0947), ICE2 (NARG2), MED26, TAF7 and EAF1 were subcloned into pFastBac HTb (Life Technologies, Carlsbad, CA) or pBacPAK8 with epitope tags and expressed singly or together with the BAC-to-BAC system (Clontech). Western blot Anti-FLAG M2 antibodies (1:2,000 dilutions, Sigma-Aldrich Corp.), anti-HA antibodies (1:2,000 dilutions, Covance, Princeton, NJ), anti-Myc antibodies (1:1,000 dilutions, Covance), anti-TAF7 antibodies (1:200 dilutions, sc-101167, Santa Cruz Biotechnology, Santa Cruz, CA), anti-ELL antibodies (1:1,000 dilutions, A301-645A, Bethyl Laboratories, Montgomery, TX), anti-EAF2 antibodies (1:1,000 dilutions, A302-502A-1, Bethyl Laboratories), anti-Rpb1 antibodies (1:2,000 dilutions, sc-899 X, Santa Cruz Biotechnology) and anti-MED1 antibodies (1:2,000 dilutions, sc-5334 X, Santa Cruz Biotechnology) were used in western blots. Mouse monoclonal anti-EAF1 antibody (1:500 dilutions) was a gift from Michael Thirman (Department of Medicine, University of Chicago). Uncropped immunoblots are shown in Supplementary Figs 8–17 . Immunoprecipitation and affinity purification Protein complexes were purified from nuclear extracts or S100 fractions of cell lines stably expressing FLAG-tagged proteins using anti-FLAG M2 agarose (Sigma-Aldrich Corp.) as described previously [45] . Briefly, nuclear extracts and S100 fractions were prepared according to the method of Dignam et al . [46] from parental HeLa cells or HEK293 FRT cells stably expressing FLAG-tagged proteins. Each of the nuclear extracts or S100 fractions was incubated with 100 μl anti-FLAG agarose beads for 2 h at 4 °C. The beads were washed five times with a 100-fold excess of a buffer containing 50 mM HEPES-NaOH (pH 7.9), 0.3 M NaCl, 0.1% Triton X-100 and 10% (v/v) glycerol, and then eluted with 100 μl of a buffer containing 0.1 M NaCl, 50 mM HEPES-NaOH (pH 7.9), 0.05% Triton X-100, 10% (v/v) glycerol and 0.25 mg ml −1 FLAG peptide. Oligo(dC)-tailed template transcription assay Transcription reactions were carried out in the presence of 20 mM HEPES-NaOH, pH 7.9/20 mM Tris-HCl, pH 7.9/60 mM KCl/2 mM dithiothreitol (DTT)/0.5 mg ml −1 BSA/1% (wt/vol) polyvinyl alcohol (average molecular weight of 30,000–70,000 Da)/3% (wt/vol) glycerol/8 U of RNasin/8 mM MgCl 2 /25 ng oligo(dC)-tailed pAd-GR220/~0.01 U Pol II and ribonucleoside triphosphates and transcription factors as indicated in the figures. In the experiments for which results are shown in Fig. 2f , reaction mixtures were preincubated for 30 min at 28 °C before the addition of ribonucleoside triphosphates. Reactions were stopped after incubation at 28 °C for the times indicated in the figure, and products were resolved on 6% polyacrylamide gels containing 7 M urea, 45 mM Tris-borate and 1 mM EDTA (pH 8.3). Generation of MEF cells ES cell line RRR660, in which the gene trapping construct pGT0lxf had been inserted into the first intron of one allele of the mouse MED26 gene, was purchased from Mutant Mouse Regional Resource Center (MMRRC) at JAX. The ES cell line was injected into blastocysts of C57BL/6 mice, and chimera mice were generated. After heterozygous mice had been generated, homozygous embryos were generated by mating heterozygous mice. The embryos were covered in PBS, and the placenta, other maternal tissues, head, limbs and all innards were removed and then homogenized with a 22-gauge syringe. MEF cells were then cultured under an atmosphere of 5% CO 2 at 37 °C in DMEM (Sigma-Aldrich Corp.) supplemented with 10% (v/v) fetal bovine serum (Invitrogen), 55 μM β-mercaptoethanol (Gibco), 2 mM L -glutamine, penicillin (10 U ml −1 ) and streptomycin (0.1 mg ml −1 ). MED26 gene trap MEF cell lines stably expressing HA-tagged MED26 wt or mutant (R61A, K62A) were generated by a Plat E retrovirus packaging system [47] . Immobilized oligo(dC)-tailed template assays A biotinylated oligo(dC)-tailed template generated from the plasmid pAd-GR220 was immobilized on Dynabeads (Life Technologies). Promoter-binding assays were performed as follows. Various combinations of proteins were incubated with 2.0 μl of Dynabeads in a reaction mixture containing 62.5 mM KCl/12.5% v/v glycerol/12.5 mM HEPES, pH 7.9/20 mM Tris-HCl, pH 7.9/0.06 mM EDTA, pH 8.0/7.5 mM MgCl 2 /0.5 mg ml −1 BSA/0.3 mM DTT/0.025% NP40 in a total volume of 60 μl. After 30 min at 28 °C, beads were collected using a magnetic particle concentrator (Life Technologies), washed three times in the same buffer without BSA and resuspended in SDS–PAGE loading buffer. Bound proteins were identified by western blot [45] . Gene expression analysis Total RNA was isolated using Isogen II (Nippon gene, Tokyo, Japan). For RT–qPCR, total mRNA was reverse transcribed using the iScript Select cDNA Synthesis Kit (Bio-Rad, Hercules, CA). The threshold cycle ( C t ) values were determined by real-time PCR reactions using Applied Biosystems StepOne Realtime PCR System and Power SYBR Green PCR Master Mix (Life Technologies) and normalized by subtracting the C t value of the GAPDH gene from the C t value of the respective gene (Δ C t = C t gene − C t GAPDH ). The relative mRNA levels were then calculated using 2 −Δ C t . Primer sequences are listed in PCR primers of Supplementary Information . ChIP assays Cells from one 10-cm dish (~1 × 10 7 ) of HEK293T cells grown to 70–80% confluence were used for each immunoprecipitation. The cells were crosslinked with 2 mM DSG Crosslinker (c1104, ProteoChem, Loves Park, IL) in PBS for 30 min and then 1% formaldehyde in PBS for 20 min at room temperature. Then, the cells were resuspended and lysed in lysis buffer (0.2 or 0.5% SDS, 10 mM EDTA, 150 mM NaCl, 50 mM Tris-HCl, pH 8.0) and they were sonicated with a Bioruptor Sonicator (Diagenode, Denville, NJ) for 15 or 30 times for 30 s at the maximum power setting to generate DNA fragments of ~150–500 bps. Sonicated chromatin was incubated at 4 °C overnight with 5–10 μg of normal IgG or specific antibodies. Specific antibodies used were as follows: MED26 (H-228, sc-48776 X, Santa Cruz Biotechnology), MED23 (A300-425A-1, Bethyl Laboratories), ICE1 (raised against bacterially expressed, His-tagged recombinant proteins of ICE1 1,865–2,266 aa), ELL (A301-645A, Bethyl Laboratories), EAF2 (A302-502A-1, Bethyl Laboratories), TAF7 (SQ-8, sc-101167, Santa Cruz Biotechnology), Rpb1 (N20, sc-899, Santa Cruz Biotechnology) and RNA Pol II CTD phospho Ser7 (Cat# 61087, Active motif, Carlsbad, CA). Then, rProtein A Sepharose (17-1279-02, GE Healthcare, Pittsburgh, PA) was added and incubated for 2 h at 4 °C. The beads were washed two times with IP buffer (20 mM Tris-HCl, pH 8.0, 150 mM NaCl, 2 mM EDTA, 1% Triton X-100), two times with high-salt buffer (20 mM Tris-HCl, pH 8.0, 500 mM NaCl, 2 mM EDTA, 1% Triton X-100), once with LiCl buffer (250 mM LiCl, 20 mM Tris-HCl, pH 8.0, 1 mM EDTA, 1% Triton X-100, 0.1% NP40 and 0.5% NaDOC) and two times with TE buffer. Bound complexes were eluted from the beads with 100 mM NaHCO 3 and 1% SDS by incubating at 50 °C for 30 min with occasional vortexing. Crosslinking was reversed by overnight incubation at 65 °C. Immunoprecipitated DNA and input DNA were treated with RNase A and proteinase K by incubation at 45 °C. DNA was purified using the QIAquick PCR purification kit (28106, Qiagen, Valencia, CA) or MinElute PCR purification kit (28006, Qiagen). Immunoprecipitated and input material was analysed by quantitative PCR. ChIP signal was normalized to total input. Three biological replicates were performed for each experiment. Primer sets are detailed in Supplementary Information . ChIP-seq and gene annotation Sequencing reads were acquired through primary Solexa image analysis. Filtered reads were then aligned to the human genome (hg19) using the Bowtie alignment tool. Only those sequences that matched uniquely to the genome with up to two mismatches and mapped to less than three locations were retained for subsequent analyses. Sequence reads for each ChIP-seq data set and its associated whole-cell extract controls were used for input. Sequence reads from triplicate or single ChIP-seq data set of ICE1 (KIAA0947) or TAF7 were used in analysis with the MACS2 peak finding program version 2.0.10, and significantly enriched regions of ChIP-seq signals were determined. Three of each data set from triplicate samples was summed up using MACS2. The significance cut-off was set to false discovery rate <1% and a fold change between 5 and 50. All other MACS parameters were left default. Genes were identified if an enriched peak region was found within ±1 kbp of the TSS of any transcript isoform of the gene. The txStart positions of the Ensembl gene annotation were used for TSS analysis. siRNA transfection HEK293T cells in six-well tissue culture plates (~1 × 10 5 cells per well) or 10-cm dishes (~2 × 10 6 cells per dish) were transfected with 50 nM siRNAs targeting human MED26 (#1, s18074; #2, s18075; #3, s18076, Ambion/Life Technologies), with 50 nM of siRNA targeting human TAF7 (ON-TARGET plus SMART pool, L-013669-00, Dharmacon, Pittsburgh, PA) or with 50 nM siGENOME NON-TARGETING siRNA Pool #2 (D-001206-14, Dharmacon) using Lipofectamine RNAiMAX Transfection Reagent (Invitrogen). Immunostaining HeLa cells grown on glass coverslips were fixed for 7 min at room temperature with 100% methanol. Then, the cells were incubated for 15 min with PBS containing 0.2% Triton X-100. After blocking cells with Tris buffered saline with Tween 20 (TBST) containing 3% BSA, the cells were incubated at room temperature with primary antibodies to coilin (ab11822, Abcam, Cambridge, UK) at 1:1,000 dilutions, MED26 (H-228, sc-48776 X, Santa Cruz Biotechnology) at 1:2,000 dilutions or ICE1 (KIAA0947) at 1:1,000 dilutions in TBST containing 3% BSA. The cells were then incubated with Alexa488-labelled goat polyclonal antibody to mouse IgG or Alexa546-labelled goat polyclonal antibody to rabbit IgG (Life Technologies), covered with a drop of VECTASHIELD (Vector Laboratories, Burlingame, CA) and then photographed with a charge-coupled device camera (DP71, Olympus, Japan) attached to an Olympus BX51 microscope. How to cite this article : Takahashi, H. et al . MED26 regulates the transcription of snRNA genes through the recruitment of little elongation complex. Nat. Commun. 6:5941 doi: 10.1038/ncomms6941 (2015). Accession codes: The ChIP-seq data are available under DDBJ sequence Read Archive, accession number DRA002712 .